The N-terminus of anUstilaginoidea virensSer-Thr-rich glycosylphosphatidylinositol-anchored protein elicits plant immunity as a MAMP 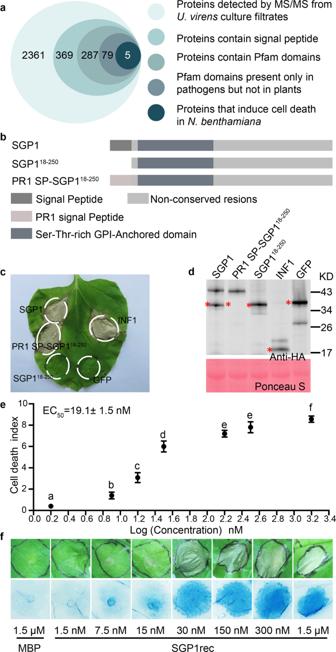Fig. 1: SGP1 is an apoplastic elicitor of cell death inN. benthamiana. aSystematic identification of SGP1 amongU. virenssecreted proteins. The numbers in circles represent proteins that met successively stringent criteria.bRegions of SGP1 examined for cell death activity.cRepresentativeN. benthamianaleaves at 5 d after inoculation withAgrobacteriumstrains carrying the indicated genes in vector pGR107. Similar results were obtained from 3 independent experiments (Supplementary Data3).dWestern blot analysis of the indicated proteins transiently expressed inN. benthamiana. The red asterisks (*) indicate the predicted protein sizes in kDa.e,fCell death induced by recombinant SGP1 protein fromE. coli. MBP protein serves as a control (MBP, as the tag in empty vector, was purified in the same way as SGP1rec). Five independent experiments were performed, with five plants in each experiment.eDetermination of purified SGP1rec EC50values in cell death-inducing activity, based on cell death index (Supplementary Fig.2). Values are means ± SD of five experiments. Different letters indicate statistically significant differences (P< 0.01; Duncan’s multiple range test).fRepresentativeN. benthamianaleaves infiltrated with purified SGP1rec (1.5 nM to 1.5 μM). Upper panel, photos directly taken at 2 days post-infiltration (dpi). Lower panel, photos taken at 2 dpi after staining with trypan blue. Many pathogens infect hosts through specific organs, such as Ustilaginoidea virens , which infects rice panicles. Here, we show that a microbe-associated molecular pattern (MAMP), Ser-Thr-rich Glycosyl-phosphatidyl-inositol-anchored protein (SGP1) from U. virens , induces immune responses in rice leaves but not panicles. SGP1 is widely distributed among fungi and acts as a proteinaceous, thermostable elicitor of BAK1-dependent defense responses in N. benthamiana . Plants specifically recognize a 22 amino acid peptide (SGP1 N terminus peptide 22, SNP22) in its N-terminus that induces cell death, oxidative burst, and defense-related gene expression. Exposure to SNP22 enhances rice immunity signaling and resistance to infection by multiple fungal and bacterial pathogens. Interestingly, while SGP1 can activate immune responses in leaves, SGP1 is required for U. virens infection of rice panicles in vivo, showing it contributes to the virulence of a panicle adapted pathogen. The ability to sense the presence of potentially infectious pathogens poses a central challenge for all multicellular organisms and forms the basis for activation of innate defense mechanisms against attempted microbial infection [1] . Plant perception of molecular determinants, known as microbe-associated molecular patterns (MAMPs) or pathogen-associated molecular patterns (PAMPs) [1] , [2] , [3] , which are conserved and characteristic of classes of microbes, can trigger basal immune responses [4] , [5] . MAMPs/PAMPs have been described for bacteria, oomycetes, and fungi. They can be peptidoglycans [6] , lipopolysaccharides [7] , glucans [8] , chitins [9] , or proteins encoded for diverse functions. Well-characterized proteinaceous MAMPs/PAMPs include flagellin [10] , EF-Tu [11] , [12] , and cold shock proteins (CSPs) [13] from bacteria, transglutaminases (TGases) [14] , cellulose-binding elicitor lectin (CBEL) [15] , and elicitins [16] from oomycetes, and xylanase EIX [17] from fungi. The necrosis and ethylene-inducing peptide 1 (Nep1)-like proteins (NLPs) [18] , [19] , [20] , [21] , [22] and glycoside hydrolase 12 protein XEG1 [23] , [24] MAMPs are both extensively distributed in bacteria, oomycetes, and fungi. Typically, small epitopes within the microbial patterns are sufficient to elicit immunogenic responses [4] , [25] , [26] . For example, a highly conserved 22-aa fragment of flagellin, flg22, is sufficient to activate immunity in Arabidopsis and other plant species [10] . An 18-aa domain of EF-Tu, elf18, is recognized as a MAMP in Brassicaceae species [11] , [12] . Pep‐13, which is conserved among Phytophthora TGases, activates defense reactions in parsley and potato [14] . However, few peptides from proteinaceous MAMPs have been identified in fungi, with the exception of 24-aa peptides of NLPs that act as MAMPs in Arabidopsis [19] . Thus, the mechanisms that allow plants to perceive pathogenic fungi and to defend against infection remain mostly undiscovered. Glycosyl-phosphatidyl-inositol (GPI)-anchored proteins (GAPs) are a class of membrane-associated proteins containing a soluble protein attached by a post-translational glycolipid modification, the GPI anchor, to the external leaflet of the plasma membrane [27] . GPI is broadly distributed among eukaryotes, including protozoa, fungi, plants, insects, and mammals, while proteins containing a GPI anchor are structurally and functionally diverse and play vital roles in numerous biological processes, as enzymes, cell surface antigens, signaling receptors, cell adhesion molecules, and migration molecules [28] , [29] . For example, the GPI-anchored proteins CD55 (or decay-accelerating factor, DAF) and CD59 are important in the regulation of the complement cascade, which protects organisms from foreign invaders and pathogens [30] . Phospholipases (PLCs) can cleave the GPI anchor and release GAPs [31] . Approximately 1% of protein-coding genes in eukaryotic genomes are likely to encode GPI-anchored proteins (GAPs) [32] . Nevertheless, the specific roles of the majority of GAPs in host–microbe interactions remain largely unknown, especially in plant pathogens. Ustilaginoidea virens (Cooke) Takah is the causal agent of rice false smut (RFS), which has recently undergone a rapid expansion to emerge as one of the most destructive rice diseases worldwide [33] , [34] . For example, in China, an estimated ~2.4 million hectares per year between 2015 and 2017 are reportedly affected by this disease [35] . RFS epidemics not only lead to yield loss but also threaten food safety due to its production of mycotoxins, including ustiloxins and ustilaginoidins [35] . This pathogen is an ascomycetous fungus that predominantly attacks rice stamen filaments, extending intercellularly along the filament base, and sometimes invades lodicules [33] , [36] , [37] , but is asymptomatic in other organs such as leaves, thus leading to its categorization as a new type of flower disease [38] . The most likely route of U. virens infection is entry into the inner space of the spikelets through the gap between the lemma and palea when rice plants are at the booting stage [39] , [40] . Given its recent emergence, the mechanisms underlying plant– U. virens interactions and how plants defend themselves against infection by this pathogen remain largely unknown. Here, we identified a MAMP, SGP1, from the causal agent of RFS, U. virens , that triggers programmed cell death in several plant species, including N. benthamiana in a BAK1-dependent manner. SGP1 belongs to the Ser-Thr-rich GPI-anchored protein family, which is widely distributed in fungi, and many homologs of which induce cell death in N. benthamiana . Plants specifically recognize a peptide comprising 22 amino acids ( S GP1 N terminus p eptide 22, SNP22) in the N terminus of the protein, which can fully activate programmed cell death, oxidative burst, and upregulation of defense-related gene expression, ultimately inducing resistance against both bacterial and fungal pathogens in rice. Notably, we show that SNP22 could elicit a stronger immunity signaling response in leaves than in panicles of rice. Moreover, using SGP1 overexpression lines, SGP1 W44A overexpression (with abolished SGP1-associated MAMP activity) lines, and SGP1-silenced lines, we found that SGP1 is required for U. virens pathogenicity during infection of rice panicles in vivo, and that it appears to activate an immune response in rice leaves. SGP1 from U. virens is an apoplastic elicitor of cell death in N. benthamiana To identify potential elicitors of plant immunity from U. virens , we identified a library of 79 putative candidate proteins based on the following characteristics: 1. Proteins were detectable by MS/MS in U. virens culture filtrates from three independent experiments; 2. Proteins were predicted to contain a signal peptide by SignalP3.0; 3. Proteins were predicted to contain Pfam domains by Pfam 31.0; and 4. The predicted Pfam domains were present only in microbes, but not in plants (i.e., rice and N. benthamiana ) (Fig. 1a and Supplementary Data 1 ). We then constructed an Agrobacterium -mediated transient expression system in N. benthamiana to assay the elicitor activity of candidates, which ultimately revealed five proteins that induced cell death in N. benthamiana leaves (Fig. 1a and Supplementary Data 1 ). A Ser-Thr-rich Glycosyl-phosphatidyl-inositol-anchored family protein (SGP1), which induced cell death in N. benthamiana and is widely distributed across fungi, was selected for further study (Fig. 1b–d and Supplementary Data 1 – 3 ). In addition, we identified a paralog of SGP1 in U. virens, which did not induce cell death in N. benthamiana (Supplementary Data 1 and 2 ). Fig. 1: SGP1 is an apoplastic elicitor of cell death in N. benthamiana . a Systematic identification of SGP1 among U. virens secreted proteins. The numbers in circles represent proteins that met successively stringent criteria. b Regions of SGP1 examined for cell death activity. c Representative N. benthamiana leaves at 5 d after inoculation with Agrobacterium strains carrying the indicated genes in vector pGR107. Similar results were obtained from 3 independent experiments (Supplementary Data 3 ). d Western blot analysis of the indicated proteins transiently expressed in N. benthamiana . The red asterisks (*) indicate the predicted protein sizes in kDa. e , f Cell death induced by recombinant SGP1 protein from E. coli . MBP protein serves as a control (MBP, as the tag in empty vector, was purified in the same way as SGP1rec). Five independent experiments were performed, with five plants in each experiment. e Determination of purified SGP1rec EC 50 values in cell death-inducing activity, based on cell death index (Supplementary Fig. 2 ). Values are means ± SD of five experiments. Different letters indicate statistically significant differences ( P < 0.01; Duncan’s multiple range test). f Representative N. benthamiana leaves infiltrated with purified SGP1rec (1.5 nM to 1.5 μM). Upper panel, photos directly taken at 2 days post-infiltration (dpi). Lower panel, photos taken at 2 dpi after staining with trypan blue. Full size image In order to determine the role of the signal peptide in SGP1 activity, we deleted this region and found that loss of the signal peptide abolished the cell death-inducing ability of SGP1 in N. benthamiana . By contrast, replacing the signal peptide of SGP1 with the pathogenesis-related protein 1 (PR1) signal peptide, resulted in complementation of cell death-inducing activity (Fig. 1c and Supplementary Data 3 ). Western blot analysis showed an extra, larger band in addition to the bands at the predicted size for SGP1 and PR1 SP-SGP1 18–250 but not at SGP1 18–250 (Fig. 1d ), suggesting that this band is likely a post-translationally modified form of SGP1. Together, these data suggested that SGP1 must be targeted to the extracellular space of N. benthamiana tissue to induce cell death. The SGP1 protein induces cell death in N. benthamiana , potato plants, and rice To further confirm that SGP1 could induce cell death in N. benthamiana , the 68 kDa recombinant protein, SGP1rec (Supplementary Fig. 1 ), was infiltrated into the mesophyll of N. benthamiana leaves in a concentration from 1.5 nM to 1.5 μM. As shown in Fig. 1e, f and Supplementary Fig. 2 , the degree of cell death increased with increasing concentrations of SGP1rec. The half-maximal effective concentration (EC 50 ) value was calculated to be 19.1 nM (Fig. 1e, f ). To examine the specificity of the host response to SGP1, we infiltrated SGP1rec into expanded leaves of various plants. SGP1rec induced localized cell death in potato ( Solanum tuberosum ), but not in tomato ( Solanum lycopersicum ), soybean ( Glycine max ), pepper ( Capsicum annum ), maize ( Zea mays ), wheat ( Triticum aestivum ), and cotton ( Gossypium hirsutum ) (Fig. 2a–g and Supplementary Data 3 ). Due to technical issues with infiltration of SGP1rec into rice leaves, rice suspension cells were instead used to determine the cell death activity of SGP1 by Evans blue staining. As shown in Fig. 2h , exposure of cells to SGP1rec resulted in a threefold increase in Evans blue signal compared with controls at 12 h after treatment, thus indicating that SGP1rec induced cell death in rice suspension cells. Together, these experiments showed that SGP1 can induce cell death in at least three different plant species. Fig. 2: Specificity of the host response to SGP1 and wide distribution of SGP1 homologs across fungal species. a – h Cell death responses in other plant species triggered by exposure to 1 μM SGP1rec or MBP control. a – g Representative leaves are shown for potato plants ( a ), tomato ( b ), soybean ( c ), pepper ( d ), maize ( e ), wheat ( f ), and cotton ( g ). Data were obtained from three independent experiments, with 10 plants of each species per experiment (Supplementary Data 3 ). Dotted circles indicate infiltration area. The plus symbol (+) indicates that the cell death phenotype was observed, and the minus symbol (−) indicates the absence of a clear cell death phenotype. h Cell death induced by SGP1rec in rice suspension cells. Cell death was quantified by detection of Evans Blue signal released from rice suspension cells (μg/g) after treatment with SGP1rec or MBP. Data were obtained from five independent experiments, with three replicates in each experiment. In box plots, whiskers indicate the minimum and maximum values, the line indicates the median, the box boundaries indicate the upper (25th percentile) and lower (75th percentile) quartiles. ** P < 0.01, two-sided t -test. i Distribution of SGP1 across fungal species. The fungal species include both plant pathogenic and non-pathogenic fungi. Left, Maximum-Likelihood phylogenetic tree of fungal species which contain the Ser-Thr-rich GPI-anchored domain, reconstructed using PhyML v3.0 based on single-copy orthologs (Supplementary Data 5 ). Right, representative hosts of the corresponding pathogens. Image credit: https://www.flaticon.com or https://icons8.com/icons . j Phylogeny of SGP1 and 123 related sequences from selected fungal species (Supplementary Data 2 and 4 ). The proteins that induce cell death in N. benthamiana are indicated by a red dot and those that do not are indicated by a gray dot. Full size image SGP1 belongs to the Ser-Thr-rich Glycosyl-phosphatidyl-inositol-anchored protein family, which is widely distributed across fungi Since SGP1 contains a distinctive Ser-Thr-rich GPI-anchored family domain, we studied the phylogenetic distribution of this protein domain in various organisms. We subsequently performed annotation of Pfam Ser-Thr-rich GPI-anchored domain (PF10342.8)-containing proteins in five plants, nine bacteria, five oomycetes, and thirty fungi (Supplementary Data 2 ). However, no proteins containing this domain were found in the plant, bacterial or oomycete species, but they were widely present in fungi, including crop pathogens such as Puccinia graminis , Fusarium solani , and Magnaporthe oryzae ; vegetable pathogens such as Botrytis cinerea and Sclerotinia sclerotiorum ; and fruit pathogens such as Valsa mali (Fig. 2i and Supplementary Data 2 , 4 , 5 ). These results suggested that Ser-Thr-rich GPI-anchored family proteins are common across fungal taxa. The Ser-Thr-rich GPI-anchored family proteins from diverse fungal species, including biotrophic, necrotrophic, and hemibiotrophic pathogens, were then tested for their ability to induce cell death using agroinfiltration in N. benthamiana . Of the 50 genes we cloned from pathogens, 18 triggered visible cell death. At least one protein each from the biotrophic pathogens Sporisorium reilianum , Ustilago maydis , and Claviceps purpurea , necrotrophic pathogens Botrytis cinerea , Valsa mali , Verticillium dahliae , and Aspergillus flavus , as well as hemibiotrophic pathogens Sclerotinia sclerotiorum , Fusarium solani , Fusarium oxysporum , and Fusarium verticillioides all induced cell death in N. benthamiana (Fig. 2j and Supplementary Data 2 , 4 ). In addition, two proteins from fungi not associated with plants could also induce cell death in N. benthamiana . Based on these results, we concluded that Ser-Thr-rich GPI-anchored family proteins from diverse pathogens were recognizable by N. benthamiana . Cell death triggered by SGP1 in N. benthamiana requires BAK1 To determine whether BAK1, a central regulator of innate immunity, participates in the induction of cell death by SGP1, virus-induced gene silencing (VIGS) constructs were used to silence BAK1. The results showed that both INF1 and SGP1-triggered cell death in TRV: EV lines (Fig. 3a and Supplementary Data 3 ), as anticipated, while both failed to trigger cell death in BAK1 -silenced plants. Western blot confirmed the successful expression of SGP1 in TRV transgenic lines (Fig. 3b ). Quantitative real-time PCR (qRT-PCR) relative expression analysis revealed that BAK1 transcripts were markedly reduced in TRV: BAK1 lines compared with TRV: EV lines (Fig. 3c ). These results suggested that BAK1 was involved in SGP1-triggered cell death in N. benthamiana . Fig. 3: Cell death triggered by SGP1 requires BAK1 but is not affected after treatment with PI-PLC or heat in N. benthamiana . a – c Cell death triggered by SGP1 requires BAK1. a SGP1-triggered cell death in TRV-silenced N. benthamiana . Representative photographs were taken at 5 days post-infiltration. Data were obtained from 3 independent experiments, each of which used 10 VIGS-silenced plants per line (Supplementary Data 3 ). The plus symbol (+) indicates a positive cell death phenotype; minus symbol (−) indicates the absence of a clear cell death phenotype. b Western blot analysis of proteins transiently expressed in VIGS-silenced N. benthamiana leaves. The red asterisks (*) indicate the predicted protein sizes. c qRT-PCR quantification of relative transcript levels of BAK1 in VIGS-silenced N. benthamiana leaves, normalized to those in TRV: EV lines, using the EF1α gene as an internal reference. Means and standard deviations obtained from three biological replicates. (** P < 0.01, two-sided t -test). d Cell death activity of SGP1rec in the presence or absence of PI-PLC, with MBP as a control. Data represent the results of three independent experiments in each of which one leaf was sampled and infiltrated from each of three plants per treatment (Supplementary Data 3 ). e Cell death response induced by heat-treated SGP1rec in N. benthamiana leaves. SGP1rec was treated under 100 °C for 10 min. Three independent experiments were performed (Supplementary Data 3 ), in each of which ten leaves were sampled per treatment. The plus symbol (+) indicates a positive cell death phenotype; minus symbol (−) indicates the absence of a clear cell death phenotype. Full size image SGP1-triggered cell death is not affected by phospholipase C treatment or heat treatment SGP1 was predicted to have the essential characteristics necessary for GPI modification. To determine whether SGP1 was modified by GPI, we performed phase partition assays to test whether SGP1 protein moved from the hydrophobic detergent phase to the aqueous phase following phosphatidylinositol-specific phospholipase C (PI-PLC) treatment. Several forms of SGP1, including potential glycosylated- or polymers of SGP1, were detected in the aqueous phase after treatment with PI-PLC, whereas little protein was detected in the aqueous phase in the absence of PI-PLC (Supplementary Fig. 3a ). An ~80 kDa band was present in the aqueous phase after PI-PLC treatment but not in the detergent phase (Supplementary Fig. 3a ), which we hypothesized could be a previously unrecognized form of SGP1 protein released from the detergent phase. These results suggested that SGP1 was modified by GPI when expressed in N. benthamiana . To test whether the GPI modification was also involved in the induction of cell death by SGP1, we next infiltrated PI-PLC into N. benthamiana leaves 24 h after Agro -infiltration (Supplementary Fig. 3b ) or co-infiltrated PI-PLC together with SGP1rec into N. benthamiana leaves (Fig. 3d and Supplementary Data 3 ). The results indicated that SGP1-triggered cell death was not affected by PI-PLC treatment. In addition, SGP1rec was still able to trigger cell death in N. benthamiana leaves even after heat treatment by boiling for 10 min (Fig. 3e and Supplementary Data 3 ). Taken together, these results demonstrated that SGP1 could function as a thermostable protein elicitor of cell death in N. benthamiana . The N terminus of SGP1 contains the elicitor-active epitope To identify the location of the SGP1 protein epitope responsible for elicitor activity, we generated truncated mutant variants of SGP1 which carried an intact signal peptide and tested them for induction of cell death by agroinfiltration in N. benthamiana . As shown in Fig. 4a and Supplementary Data 3 , the region containing residues 22–120, corresponding to the Ser-Thr-rich GPI-anchored domain of SGP1, fully triggered cell death in N. benthamiana leaves. Western blot showed that the bands corresponding to the predicted molecular weights were detectable in all of the truncated SGP1 variants (Fig. 4b ). These results indicated that the elicitor-active epitope likely resides in the N terminus of SGP1. In addition, heterologous expression of the Ser-Thr-rich GPI-anchored domains of SGP1 homologs from U. virens , C. purpurea , or F. solani also induced cell death in N. benthamiana (Fig. 4c and Supplementary Data 3 ), thus indicating the participation of this conserved domain in triggering cell death. Moreover, the SGP1 N-terminus protein (SNPrec) was found to retain its ability to induce cell death even after heat treatment (Supplementary Fig. 4 ). Furthermore, sequence alignment of the full length of Ser-Thr-rich GPI-anchored proteins showed that the N-terminal sequences are more conserved than the C terminus, indicating a potentially conserved epitope located in the SGP1 N terminus (Supplementary Fig. 5 and Supplementary Data 4 ). Western blots (Fig. 4b ) showed that the protein abundance of SGP1 1–107 was lower than that of SGP1 1–120 , suggesting that the low abundance of SGP1 1–107 may be related to its failure to induce cell death in N. benthamiana . Fig. 4: A 22 amino acid fragment in the N terminus of SGP1 is sufficient to mediate cell death in N. benthamiana . a – c Regions of SGP1 examined for cell death activity. Plus symbol (+), cell death phenotype; minus symbol (−), no clear cell death phenotype. Cell death phenotypes were recorded at 5 dpi. a Regions of SGP1 were examined for cell death activity by agrobacterium-mediated transient expression. Similar results were obtained from four independent experiments, with 10 plants per strain in each experiment (Supplementary Data 3 ). b Western blot analysis of SGP1 and truncated mutant variants transiently expressed in N. benthamiana leaves. The red asterisk (*) indicates the predicted protein sizes. c Regions of SGP1 examined for cell death activity in N. benthamiana by infiltration with 1 μM purified SGP1 variants from E. coli . Similar results were obtained from three independent experiments (Supplementary Data 3 ). d Sequence logos indicating the level of conservation for each residue of SNP22 region in GPI-anchored proteins that trigger cell death from plant-associated fungi. Sequence logos were constructed with Geneious R11 (Supplementary Data 6 ). The character and size of each logo represent the proportion of homologs with the amino acid at that specific site. e , f Cell death triggered by expression of recombinant SNP22 homolog proteins from other fungi and alanine-substituted versions of SNP22rec. e Sequence alignment and cell death-inducing activity of the SNP22 region of SGP1 homologs that can induce cell death. The homologous sequences of SNP22 from other fungi, including four amino acids flanking either terminus (Supplementary Data 7 ), were expressed in E. coli . Vm , KUI59516 ( Valsa mali ); Bc , Bcin01p05310.2 ( Botrytis cinerea ); Ss , EDO01950 ( Sclerotinia sclerotiorum ); Cp , CCE31100 ( Claviceps purpurea ); Fv , FVEG_00876T0 ( Fusarium verticillioides ); Fs , NechaP98847 ( Fusarium solani ); Vd , VDAG_JR2_Chr3g03370a-00001 ( Verticillium dahliae ); Mo , MGG_04599T0 ( Magnaporthe oryzae ). Three independent experiments were performed, using 10 plants for each SNP22 homolog (Supplementary Data 3 ) in each experiment. f Representative photos of cell death triggered by SNP22rec variants with single alanine substitutions at the indicated residues. Similar results were obtained from three independent experiments, with five plants per protein in each experiment (Supplementary Data 3 ). Full size image A 22 amino acid peptide (SNP22) occurring in diverse fungal species is sufficient to induce ROS production and cell death in N. benthamiana To further identify the minimal immunogenic epitope within SGP1, nested peptides covering the entire SGP1 protein sequence were synthesized and tested for their abilities to trigger r eactive o xygen s pecies (ROS) production in N. benthamiana leaf disks (Fig. 5a ). Two overlapping peptides of SGP1, i and p, spanning residues I16 to S45 and D23 to G53, respectively, clearly showed the ability to induce an ROS burst. These peptides overlapped from D23 to S45 (DPIYTPNSGETIDAGAPYTVTWS, peptide 1, Fig. 5d ), suggesting that this fragment constitutes the core of the immunogenic activity of SGP1. Synthetic peptides progressively shortened by C-terminal or N-terminal deletions were further analyzed to determine the minimal length required for immunogenic activity (Fig. 5b–d ). The EC 50 value determined for SNP22 was similar to that of peptide 1, while the EC 50 values of SNP21 and SNP20 were nearly twice that of SNP22. Peptide 3, which lacks W44, and peptide 6, which lacks I25, did not induce ROS production even at 10 μM concentrations (Fig. 5d ). The total ROS production triggered by SNP22 was also nearly twofold greater than that of SNP21 and SNP20 (Fig. 5c ). These results indicated that the 22 amino acid peptide was sufficient to induce ROS production, and the minimal peptide capable of inducing an ROS burst in N. benthamiana could be as small as 20 amino acids. Fig. 5: A 22 amino acid peptide (SNP22) of SGP1 is sufficient to induce ROS production in N. benthamiana . a Schematic representation of synthetic peptides (30-mer peptides, a–r) covering wild-type SGP1. b ROS production dynamics induced by 1 μM peptides of SNP22 and SNP22 W44A in N. benthamiana leaf discs. 100 nM flg22 and buffer served as positive and negative controls, respectively. ROS production was measured with a luminol-based assay. Leaf discs from 3- to 4-week-old N. benthamiana plants were incubated with the indicated peptides, and the luminescence was expressed as relative light units (RLU). Values represent means ± SEM of three leaf disks, each sampled from a different plant and tested in parallel. c Dose–response curves of total ROS production induced by SNP22, SNP21, SNP20, SNP22 I25A , or SNP22 W44A peptides in N. benthamiana leaf discs. Values represent the means ± SEM of three independent experiments, each of which used three leaf disks per treatment. d Summary of EC 50 values determined from dose–response curves based on total ROS production. Peptide names and sequences are indicated on the left. EC 50 values of each peptide are shown on a logarithmic scale on the right. Values represent the means ± SEM of three independent experiments, with three leaf disks per treatment used in each experiment. No activity could be detected with peptides denoted by red triangles at 10 μM. Vm , KUI59516 ( Valsa mali ); Bc , Bcin01p05310.2 ( Botrytis cinerea ); Ss , EDO01950 ( Sclerotinia sclerotiorum ); Cp , CCE31100 ( Claviceps purpurea ); Fv , FVEG_00876T0 ( Fusarium verticillioides ); Fs , NechaP98847 ( Fusarium solani ); Vd , VDAG_JR2_Chr3g03370a-00001 ( Verticillium dahliae ); Mo , MGG_04599T0 ( Magnaporthe oryzae ). Full size image To test whether SNP22-like peptides of GPI-anchored protein from other fungi harbor MAMP activity, we next analyzed the immunogenic potential of synthetic peptides that represented other fungi-derived sequences orthologous to SNP22 of UvSGP1. The results showed that FsSNP22, CpSNP22, and SsSNP22 all induced ROS production, while VmSNP22, BcSNP22, and FvSNP22 did not, even at 10 μM concentrations (Fig. 5d ). The synthetic peptides were also tested for their cell death-inducing activity in N. benthamiana leaves and only CpSNP22 was found to induce an obvious cell death phenotype (Supplementary Fig. 6 and Supplementary Data 3 ). The inconsistency in the induction of ROS production and the induction of cell death between the synthetic peptides and their corresponding recombinant full-length proteins may be caused by differences in stability, folding, or conformation [15] , [17] , [41] . To address this issue, we then used recombinant SNP22 (SNP22rec) to test the ability of this peptide to trigger cell death and found that SNP22rec could indeed induce cell death in N. benthamiana (Fig. 4c ). Furthermore, a minimal 21 amino acid region of this recombinant protein (SGP1 24-44 rec) was enough to induce cell death (Fig. 4c and Supplementary Data 3 ). Then, to investigate whether this 22 amino acid region in other fungi could also induce cell death, we tested homologous recombinant SNP22 proteins (plus 4 flanking residues at each terminus) from other plant-associated fungi. These experiments showed that BcSNP22rec, ScSNP22rec, FsSNP22rec, and CpSNP22rec could all induce cell death in N. benthamiana (Fig. 4d, e and Supplementary Data 3 , 6 , 7 ), indicating that the cell death-inducing activity of this region is conserved across SGP1 homologs. To determine which amino acids were required for MAMP activity of the SNP22 region, we determined the cell death-inducing activity of SNP22rec variants carrying single alanine substitutions at each of the 22 residues (Fig. 4f and Supplementary Data 3 ). The results suggested that I25, Y26, I34, G37, Y40, T41, V42, and W44 residues are required for its induction of programmed cell death, among which I25, I34, G37, V42, and W44 were the most conserved residues (Fig. 4d, f and Supplementary Data 3 , 6 ). In addition, analysis of ROS production triggered by synthetic SNP22 variants with single alanine substitutions at the conserved amino acids or at residues found to be necessary for inducing cell death, suggested that I25, Y26, I34, G37, Y40, V42, and W44 residues are required for SNP22 activation of ROS production (Fig. 5b–d ). These results suggested that the I25, Y26, I34, G37, Y40, V42, and W44 residues may be required for receptor recognition of SGP1 to induce cell death and ROS production. Next, to test whether the SNP22 fragment determines the full activity of SGP1 in inducing cell death and ROS production, we generated the recombinant SGP1 mutants SGP1 I25A rec and SGP1 W44A rec and found that neither SGP1 I25A rec nor SGP1 W44A rec was able to induce cell death or ROS production (Supplementary Fig. 7 and Supplementary Data 3 ). Thus, the alanine substitutions in I25 or W44, which abolished the elicitor ability of SNP22rec, also abolished the activity of the full-length SGP1rec, indicating that the SNP fragment is the determinant of SGP1 elicitor activity. Taken together, we can infer that SNP22 could serve as a minimal immunogenic epitope of SGP1 in MAMP activity. SNP22 triggered the induction of disease resistance in N. benthamiana and rice To determine whether SNP22 triggers immunity in non-host N. benthamiana , we firstly determined whether SNP22 pretreatment could enhance the resistance of N. benthamiana to Phytophthora parasitica var nicotianae . We found that lesion diameter and relative P. parasitica biomass in N. benthamiana leaves were significantly reduced in plants pretreated with SNP22 peptide compared to mock and SNP22 W44A pretreatment (Fig. 6a–c ). There were no detectable, direct effects of SNP22 on P. parasitica growth on plates, indicating that SNP22 peptides did not exert any direct toxicity against P. parasitica (Supplementary Fig. 8 ). We then investigated whether SNP22 could induce defense responses other than disease resistance. Compared with control and SNP22 W44A peptides, the relative expression of defense-related genes and ROS accumulation were enhanced after treatment with SNP22 peptide (Supplementary Fig. 9 ). Taken together, these results indicated that SNP22 triggered the activation of a canonical defense response signal cascade and disease resistance in N. benthamiana . Fig. 6: SNP22 triggers induction of disease resistance in N. benthamiana and rice. N. benthamiana leaves, rice panicles, and rice leaves were pretreated with 1 μM of the indicated peptide for 24 h before pathogen inoculation. Buffer served as a mock treatment. In box plots, whiskers indicate the minimum and maximum values, line indicates the median, the box boundaries indicate the upper (25th percentile) and lower (75th percentile) quartiles. (** P < 0.01 compared with Mock, two-sided Dunnett’s test). a – c Induction of disease resistance to P. parasitica var nicotianae in N. benthamiana . a Lesions were assessed under UV light and representative photographs were taken at 48 h post inoculation (hpi). b Statistical analysis of lesion diameters. Data was obtained from six independent experiments, each of which tested five leaves for each treatment. c Relative biomass of P. parasitica in N. benthamiana leaves quantified by qPCR analysis of genomic DNA and normalized to mock treatment. Values from five biological replicates were shown, which include three technical replicates for each biological replicate. d – f Induction of disease resistance to M. oryzae in rice leaves. d Representative photographs were taken at 7 dpi. e Quantification of lesion types per 5 cm leaf strip. See Methods for description of lesion types. Values represent the means ± SD of five independent experiments, each of which used 10 leaves for each treatment. f Relative biomass of M. oryzae in rice leaves, quantified by qPCR analysis of genomic DNA and normalized to mock treatment. Values from five biological replicates were shown, which include three technical replicates for each biological replicate. g – i Disease resistance to U. virens in rice panicles. g Representative photographs were taken at 30 dpi. h Quantification of false smut balls per panicle. The data were collected from five independent experiments, with a total of at least 44 panicles per line. i Relative biomass of U. virens in rice spikelets, measured by qPCR analysis of genomic DNA and normalized to mock treatment. Values from five biological replicates were shown, which include three technical replicates for each biological replicate. Full size image To further evaluate the biological significance of the SNP22 region in the cognate host, we determined if resistance was successfully induced against Magnaporthe oryzae in leaves and against U. virens in rice panicles. As shown in Fig. 6d–f , M. oryzae lesions and biomass on rice leaves were significantly reduced following SNP22 pretreatment compared to mock or SNP22 W44A pretreatment. Nevertheless, compared with mock or SNP22 W44A peptide pretreatment, no obvious differences could be detected in the number of false smut balls per panicle or in the relative U. virens biomass after SNP22 pretreatment (Fig. 6g–i ). Taken together, these results indicated that SNP22 could trigger the induction of disease resistance in rice leaves to M. oryzae but not in rice panicles to U. virens . Responses to SNP22 differ between leaves and panicles of rice To assess whether SNP22-induced plant defense differs between leaves and panicles, we examined the activation of the defense-related gene, mitogen‐activated protein kinase (MAPK), and ROS production in rice leaves and panicles. As shown in Fig. 7a, b and Supplementary Fig. 10a , the activation of pattern-triggered immunity (PTI) marker gene Os04g10010 [42] , salicylic acid (SA) responsive gene PR10 , together with ethylene (ET) responsive gene phenylalanine ammonia lyase ( PAL ), was stronger in leaves than in panicles after treatment with SNP22 peptide, compared with that in SNP22 W44A -treated plants. MAPK phosphorylation levels (Fig. 7c ) and ROS production (Supplementary Fig. 10b ) increased significantly in rice leaves but were not significantly changed in rice panicles after treatment with SNP22 peptide. To further assess the differences in immunity induced by SNP22, we next performed RNA-seq. As shown in Fig. 7d , overall, PTI marker, SA-, ET-, jasmonic acid (JA)-, and abscisic acid (ABA)-related defense genes were induced after SNP22 treatment. In addition, the fold changes in the upregulation of most defense-related genes were substantially higher in leaves than in panicles, although with some exceptions such as NPR1, OsACS65, OsERF, OsLOX , and OsCytP450 . Similar transcriptional patterns of Os 04g10010, PR10, and PAL were observed in qRT-PCR assays, thus validating the RNA-seq results (Fig. 7a, b and Supplementary Fig. 10a ). Taken together, we infer that SNP22 induced stronger responses in rice leaves than in panicles. Fig. 7: Immune responses triggered by SNP22 in rice leaves and panicles. a – c Rice leaves and panicles were treated with either 1 μM SNP22 peptide, SNP22 W44A peptide, or chitin (hexa- N -acetylchitohexaose). a , b Relative induction of defense-related gene expression in rice leaves and panicles triggered by the indicated elicitors. Defense-related gene expression was normalized to that of mock at each time points after treatment. Rice actin served as an internal reference. Values represent the means ± SEM of three biological replicates. c MAPK activation in rice leaves and panicles triggered by elicitors. The phosphorylation level of MAPK detected by immunoblot with anti-phospho-p44/42 MAPK (Erk1/2) antibody. d Transcriptome analysis. The relative gene expression was normalized to those of mock treatment at each time point post-treatment. Heatmap was shown based on lg values of the fold change. Cyan color, downregulation; red color, upregulation. e – h Disease resistance to X. oryzae pv. oryzae in rice leaves and to B. glumae in rice panicles triggered by the indicated elicitors. Rice leaves and panicles were pretreated with either 1 μM SNP22, SNP22 W44A , or chitin 24 h before pathogen inoculation. Symptoms were assessed at 7 dpi. Three independent experiments were performed, and ten leaves or ten panicles were used for each experiment. e Representative photographs of symptoms on rice leaves caused by X. oryzae pv. oryzae . f Lesion lengths. Values represent the means ± SD of three independent experiments, with ten leaves in each experiment (** P < 0.01 compared with Mock, two-sided Dunnett’s test). g Representative photographs of disease symptoms on rice panicles caused by B. glumae . h Disease severity in rice panicles, evaluated as described in the “Methods” section. Values represent the means ± SD of three independent experiments, with 10 panicles per treatment in each experiment (** P < 0.01 compared with Mock, two-sided Dunnett’s test). Full size image To further confirm the differences in SNP22-triggered resistance between rice leaves and panicles, we also tested SNP22-mediated resistance to rice pathogens Xanthomonas oryzae pv. oryzae (Xoo) and Burkholderia glumae , which causes bacterial leaf blight and bacterial panicle blight in rice, respectively. As shown in Fig. 7e–h , pretreatment with SNP22 led to reduced disease symptoms in leaves caused by Xoo , but not in panicle symptoms caused by B. glumae . Pretreatment with SNP22 W44A showed no impact on disease symptoms caused by either pathogen. These results suggested that SNP22 appeared to induce an effect in which rice leaves exhibited resistance to pathogen infection while panicles did not. To examine whether the unequal immune response between rice leaves and panicles triggered by SNP22 pretreatment is a general phenomenon, we examined the immune responses triggered by chitin in both organs. We observed that defense-related genes, MAPK, and ROS production were activated in both leaves and panicles after treatment with chitin, but these markers were not enhanced in either leaves or panicles after pretreatment with SNP22 W44A (Fig. 7a–c and Supplementary Fig. 10 ). In addition, pretreatment with chitin resulted in a comparable reduction in disease symptoms in both leaves (caused by Xoo) and panicles (caused by B. glumae ) (Fig. 7e–h ). Collectively, these results suggested that the unequal immune response we observed between rice leaves and panicles triggered by SNP22 pretreatment does not appear to be a general phenomenon associated with exposure to different MAMPs. SGP1 is required for U. virens pathogenicity during rice panicle infection, but it appears to induce immunity during U. virens challenge of rice leaves To determine the biological role of SGP1 during U. virens infection, we analyzed the expression patterns of SGP1 during different infection stages. The upregulation of SGP1 during the early infection stages (Fig. 8a ) suggested the potential involvement of SGP1 in U. virens infection. Next, we obtained SGP1- silenced transformants (ST-1 and ST-7), and SGP1 overexpression (OT-4 and OT-10) or SGP1 W44A overexpression (OTm-15 and OTm-25 -with abolished SGP1-associated MAMP activity) transformants in U. virens . U. virens lines expressing GFP served as transgenic controls. The relative transcript and protein levels of SGP1 in U. virens transformants were confirmed by qRT-PCR or western blot, respectively (Fig. 8b, c ). All transformants showed normal filamentous growth, conidial morphology, and hyphal morphology compared with WT or the GFP transgenic control (Supplementary Fig. 11 ). However, compared to WT and GFP strains, the number of false smut balls per panicle and the relative pathogen biomass in the two SGP1-silenced transformants were significantly reduced, while those caused by transformants overexpressing SGP1 or SGP1 W44A were increased (Fig. 8d–f ). These results indicated that SGP1 is required for pathogenicity of U. virens during infection of rice panicles. Fig. 8: Involvement in pathogenicity and elicitor function of SGP1 during U. virens infection of rice panicles and challenge of rice leaves. a The relative expression of SGP1 during different stages of infection. SGP1 expression was normalized to its expression level prior to inoculation (0 hpi) using Tubulin as an internal reference. hpi, hours post inoculation; dpi, days post inoculation. Values are the means ± SEM of three biological replicates. The different letters indicate statistically significant differences ( P < 0.05) as measured by Duncan’s multiple range test. b Relative transcript levels of SGP1 in different U. virens transgenic lines. The transcript levels were measured by qRT-PCR and normalized to those in the WT strain using Tubulin as an internal reference. ST, SGP1- silenced transformants of U. virens ; OT, SGP1 overexpression transformants of U. virens ; OTm, SGP1 W44A overexpression transformants of U. virens . Values are the means ± SEM of three biological replicates. (** P < 0.01; two-sided t -test). c Western blot analysis of SGP1 and SGP1 W44A in U. virens WT and transgenic lines with anti-GFP antibody. d – f Pathogenicity phenotypes of transgenic U. virens lines and WT. In box plots, whiskers indicate minimum and maximum values, line indicates the median, the box boundaries indicate the upper (25th percentile) and lower (75th percentile) quartiles. d Representative photographs of disease symptoms on rice panicles. e Quantification of the number of false smut balls per panicle. Data were collected from five independent experiments, with a total of at least 31 panicles per line. (* P < 0.05; ** P < 0.01 compared with WT, two-sided Dunnett’s test). f Relative U. virens biomass in infected spikelets, measured by qPCR of genomic DNA and normalized to WT. Values from five biological replicates were shown, which include three technical replicates for each biological replicate. (** P < 0.01 compared with WT, two-sided Dunnett’s test). g Relative induction of PR10 transcription in rice leaves and panicles at 12 hpi. The induction of PR10 expression in U. virens -inoculated rice was normalized to that in mock-inoculated rice, with Actin serving as an internal reference. Values are the means ± SEM of three biological replicates. (** P < 0.01; * P < 0.05; two-sided t -test). Full size image To determine whether SGP1 is recognized by rice during U. virens challenge, activation of PR10 gene expression was determined in both leaves and panicles at 12 hpi with U. virens transgenic lines or controls. The results showed that the U. virens WT strain could induce clearly unequal responses in leaves versus panicles of rice, with an approximately 50-fold increase in PR10 expression in rice leaf tissues but only about 10-fold increase in panicles (Fig. 8g ). Compared to the WT and GFP transgenic line, the activation of PR10 in leaves was significantly increased in response to OT-4 and OT-10 lines but decreased in response to OTm-15 and OTm-25 lines. These results indicated that SGP1 may have a role in activating PR10 in rice leaves during U. virens challenge. Unlike the triggering of PR10 activation in response to OT-4 and OT-10 lines compared to WT strain in rice leaves, U. virens -induced PR10 activation was lower in response to OT-4 and OT-10 lines compared to WT and GFP transgenic lines in panicles (Fig. 8g ). These results indicated that SGP1 does not appear to induce the activation of PR10 in panicles during U. virens infection. Compared to WT and GFP transgenic lines, the activation of PR10 in panicles is significantly increased in response to ST-1 and ST-7 lines but decreased in response to OTm-15 and OTm-25 lines, similar to the response in leaves. These results suggested that SGP1 may also potentially contribute to suppressing PR10 activation during infection. Taken together, these results suggested that SGP1 appears to activate an immune response in rice leaves, whereas it contributes to U. virens’ virulence during infection of rice panicles. Some pathogens infect only a specific organ or set of organs, and this organ-specific innate immunity has been well-documented in mammals. Plant pathogens are also reported to infect their hosts through specific organs, such as U. virens , suggesting that different organs may exhibit variation in their inherent capacity to resist invasion. Here, we identified the thermostable proteinaceous MAMP, SGP1, a Ser-Thr-rich GPI-anchored family protein that is widely distributed across fungal taxa. Moreover, a minimal peptide of 22 amino acids in the N terminus constitutes the immunogenic epitope of SGP1, the detection of which by a rice plant host results in an unequal, and distinctly stronger response by leaves than panicles. Notably, we found that during U. virens infection of rice in planta , SGP1 is required for U. virens infection of rice panicles, but appears to activate immunity in rice leaves. GPI-anchored proteins are structurally and functionally diverse and play vital roles in numerous biological processes [28] , [29] . In mammals, prion protein (PrP), a widely expressed and conserved GPI-anchored protein, causes a neurodegenerative disease when misfolded variants accumulate in cells [43] , [44] , [45] . In plants, GPI-anchored proteins are required for both development and immunity signaling. For example, LORELEI (LRE), which encodes a putative GPI-anchored surface protein, together with FERONIA, jointly function in pollen tube reception [46] . In the human pathogen Candida albicans , the GPI-anchored protein CaEcm33p is required for cell wall integrity, morphogenesis, and virulence [47] . The function of GPI-anchored proteins in plant pathogenic fungi has only recently been reported. The Aspergillus flavus GPI-anchored protein encoded by ecm33 participates in growth, development, aflatoxin biosynthesis, and maize infection [48] . In our study, we showed that SGP1 contrastingly functions as a recognizable MAMP, triggering innate immunity in rice leaves, but is required for U. virens pathogenicity during infection of panicles. The amino acids in SNP22rec required for triggering cell death are also required for full activation of the ROS burst by SNP22 peptide (Figs. 4 and 5 ). It is possible that SNP22 is recognized by one receptor that initiates both signaling outcomes. The minimal peptide for triggering cell death in N. benthamiana is 21 amino acids (P24-W44), while the minimal peptide for triggering ROS production is 20 amino acids (I25-W44). Deletion of the D23 and P24 residues from SNP22, to create SNP20, resulted in impaired ability to induce cell death, whereas single alanine substitutions at either residue did not attenuate SNP22 cell death-inducing activity, indicating that neither D23 nor P24 are likely receptor binding sites. It is also possible that the attenuation of SNP20-activated ROS production compared to SNP22 may be a function of its lower stability in the apoplast. Since SNP20 leads to ROS production but not cell death in N. benthamiana , it is possible that D23 to P24 may serve as structural components that maintain a MAMP configuration that triggers cell death. In addition, cell death triggered by SNP22 raises the issue that induction of cell death is not restricted to ETI signaling but can also occur as part of a PTI response. Typically, ETI is associated with cell death and systemic acquired resistance, while PTI is not. However, SGP1, together with the MAMPs CBEL, EIX, XEG1, and harpins all induce cell death in plants [23] , [49] , [50] , [51] , [52] , indicating that programmed cell death is not exclusive to ETI, and that the distinction between PTI and ETI signaling may be blurry. Organ-specific regulation of innate immunity has been described in mammals and involves complex processes with multiple contributing factors that potentially control the responsiveness of tissues or organs to MAMPs. Organ-specific responses may be dependent on differences in the threshold for receptor activation related to differences in the organ- or tissue-specific expression profiles of pattern recognition receptors (PRR), which enables different degrees of cellular-level regulation of their respective tissue microenvironments. In addition, the expression of negative regulators of TLRs is reported to vary between different organs, and ultimately these microenvironment factors converge so that TLR signaling is modulated in an organ-specific manner [53] , [54] . Many phytopathogenic fungi are commonly reported to infect their hosts through specific organs [55] . Organ- or tissue-specific immunity has been reported in plants, although the mechanisms are far from clear. Dirk et al . reported organ-specific defense responses induced by Colletotrichum graminicola in maize, including production of antimicrobial flavonoids and differential expression of defense- and stress-related genes [56] . Arabidopsis root tissues have the capacity to activate immune responses triggered by flg22 [57] , [58] . However, significant differences have been found in the intensity of these responses and in the expression of the FLS2 receptor across various root tissues, potentially due to the density of receptor distribution [59] . In our study, we observed a phenomenon in which SNP22 appears to induce a stronger response in leaves compared to panicles. In vivo experiments with transgenic U. virens lines demonstrated that SGP1 induces immunity in rice leaves but not in rice panicles during pathogen challenge of rice. By contrast, chitin triggered comparable defense responses in both rice leaves and panicles, indicating that the differences in SGP1 MAMP activity in rice are possibly organ-specific. However, we cannot rule out that any differences in penetration between MAMPs might contribute to the differences in the generality of the response. Further, we provide the caveat that potential differences in penetration by exogenously applied SNP22 could contribute to the differences in response between leaves and panicles, and that exogenous application may not perfectly replicate the distribution of the elicitor during infection. It warrants consideration that the stronger immune response in rice leaves compared to panicles triggered by this MAMP may potentially correlate with the adaptation of U. virens to panicle instead of leaf infection. Differences in MAMP-triggered immunity between organs may thus be one possible contributing factor to organ-specific specialization by pathogens. It is also possible that some pathogens have evolved organ-specific virulence factors that drive their specialized pattern of infection, thus organ-specific virulence may be an alternative explanation for organ-specific differences in infection by some pathogens. However, SGP1 is widely distributed in fungi, and among those plant pathogens that carry it, not all use an organ-specific manner of infection, which thus suggests that pathogens may evolve different strategies to escape host immune recognition or modulate host immunity. Further investigation of the molecular mechanisms of receptor recognition of SGP1 as a MAMP, as well as modulation of plant immunity by SGP1 as a virulence factor, will improve our understanding of specialized pathogens with organ-specific manners of infection. LC–MS/MS analysis of secreted proteins from U. virens LC–MS/MS analysis was performed by Beijing Bangfei Bioscience & Technology Co., Ltd. Specifically, 10-day-old U. virens culture supernatants were collected and filtered through a 0.22-µm polyvinylidene fluoride membrane (Millipore). Proteins were precipitated overnight at 4 °C by adding 20% TCA. Then the samples were centrifuged for 15 min at 15,000 × g at 4 °C. Cold acetone was added to the resultant pellets, and proteins were precipitated for 30 min at 4 °C, followed by centrifugation as above. The wash step was repeated once. The protein precipitates were air-dried for 1–3 min and dissolved in a buffer containing 8 M Urea, 100 mM Tris-HCl (pH 8.0), and 1× protease inhibitor cocktail (Roche) by incubating at 4 °C overnight. Proteins were harvested by centrifuging at 10,000× g at 4 °C for 3 min. The proteins were digested by trypsin (Promega) followed by analysis with the Orbitrap Fusion Lumos mass spectrometer (ThermoFisher Scientific, Waltham, MA, USA) coupled with a nano high-performance liquid chromatography system (UltiMate 3000 LC Dionex; ThermoFisher Scientific). The peptides were loaded onto a C18-reversed-phase column (3 μm C18 resin, 100 μm × 20 mm) and separated on an analytical column (1.9 μm C18 resin, 150 μm × 120 mm; Thermo Fisher Scientific) using mobile phase A: 0.5% formic acid /H 2 O and B: 0.5% formic acid/acetonitrile at a flow rate of 300 nL/min, using a 150 min gradient. Peptide identification was performed with the SEQUEST search engine of Proteome Discoverer 2.1 (Thermo Fisher Scientific) software using uniport- U. virens sequences downloaded from Uniprot (UP000027002) with the false discovery rate for peptides and proteins set to 0.01. The proteins and the peptides that met the successively stringent criteria mentioned in the results are shown in Supplementary Data 1 . Bioinformatics Signal peptides were identified by the SignalP 3.0 server ( http://www.cbs.dtu.dk/services/SignalP-3.0/ ). Protein domains were predicted by Pfam ( https://pfam.xfam.org/ ). For the phylogenetic tree of fungal species, the orthologous proteins between species were predicted by OrthoFinder v 2.2.6 [60] with default settings. Pairwise sequence similarities were calculated by performing all-against-all BLASTP comparisons with an E -value cutoff of 1e−5. Orthologous groups that contained only one gene for each species were selected to construct the phylogenetic tree of fungal species (Supplementary Data 5 ). Multiple sequence alignments were performed using the ClustalW2 program with default parameters. Maximum-likelihood phylogenetic dendrograms were constructed using PhyML v3.0 [61] and graphically viewed using MEGA 6 ( www.megasoftware.net ) [62] . The phylogenetic tree of proteins that contain the GPI-anchored domain (Supplementary Data 2 ) was constructed with Geneious R11 using the neighbor-joining method. Sequences of different fungi, bacteria, oomycetes, and plants were downloaded from Ensembl Genomes ( https://ensemblgenomes.org ). Cartoons were downloaded from the website https://www.flaticon.com or https://icons8.com/icons . GPI modification was predicted by the programs PSORT ( https://wolfpsort.hgc.jp/ ), PredGPI ( http://gpcr.biocomp.unibo.it/predgpi/pred.htm ), and big-PI Plant Predictor ( https://mendel.imp.ac.at/gpi/cgi-bin/gpi_pred_plants.cgi ). Plasmid construction and preparation A mixture of cDNAs from U. virens collected at different infection stages was used as a PCR template to amplify the coding sequences of U. virens genes using Phanta Super-Fidelity DNA Polymerase (P501-d1, Vazyme). Genes were cloned into a vector based on homologous recombination technology using the Vazyme ClonExpress II One Step Cloning Kit (C112, Vazyme). The primers and constructs used in this study are listed in Supplementary Data 8 and 9 , respectively. For Agrobacterium -mediated transient expression in N. benthamiana , the coding sequences of U. virens secreted proteins were separately cloned into the binary PVX vector pGR107, which adds a C-terminal 3*HA tag to the proteins. pGR107:GFP and pGR107:INF1 plasmid constructs served as negative and positive controls, respectively. For expression of the protein in E. coli , mature sequences encoding SGP1 or the mutant forms of SGP1 were cloned to the pHMTc vector, which contains an N-terminal His tag and MBP protein. For expression of the protein in U. virens , sequences encoding SGP1 or SGP1 mutants were cloned into the pKD1-GFP vector, which contains a C-terminal GFP tag. Agrobacterium and protein/peptide infiltration assays Agrobacterium -mediated transient expression assays were performed to test the cell death-inducing activity of proteins. Genes cloned into the pGR107 vector were transformed into Agrobacterium cells and then infiltrated into N. benthamiana leaves using a needleless syringe at a concentration of 0.5 OD. Agrobacterium strains carrying GFP and INF1 pGR107 constructs were infiltrated in parallel as negative and positive controls, respectively. For protein infiltration assays, the protein was expressed and purified from E. coli strain Rosetta using Ni-NTA Superflow resin (Qiagen) following the manufacturer’s instructions. Protein was first adjusted to the appropriate concentration and then infiltrated into plant leaves of different species using a needless syringe. SGP1 protein solutions ranging from 1.5 nM to 1.5 μM were infiltrated into the leaves of N. benthamiana . MBP protein expressed from the empty vector served as a negative control. Protein solutions (1 μM) were also infiltrated into the leaves of different plants. Photos were taken at 2 dpi for potato plants ( Solanum tuberosum ) and at 7 dpi for tomato ( Solanum lycopersicum ), pepper ( Capsicum annum ), maize ( Zea mays ), wheat ( Triticum aestivum ), soybean ( Glycine max ), and cotton ( Gossypium hirsutum ) plants. For the peptide infiltration assays, peptides were purchased from Synpeptide Co. and Genscript Inc. Peptides were first dissolved in DMSO to obtain a 10 mM stock solution and then diluted with distilled water to different concentrations before infiltration into N. benthamiana leaves. Western blot analysis Protein extraction buffer (10 mM Tris/Cl [pH 7.5], 150 mM NaCl, 0.5 mM EDTA, 0.5% NP-40) supplemented with protease inhibitor cocktail (Roche) was used for protein extraction from mycelia and plant materials. Protein samples of U. virens mycelia from the WT strain and the overexpression transformants were collected 7 days after culturing in potato sucrose (PS) liquid medium. Western blot analysis was performed with the eBlot™ L1 Protein Transfer System (GenScript) and Odyssey (Li-COR) detection system with IRDye 800CW Goat anti-Mouse IgG(H + L) antibody (926-32210, LI-COR,1:10000). Chemiluminescence detection in Fig. 4b was carried out with Horseradish Peroxidase (HRP)-conjugated Anti- HA antibodies (26183-HRP, Thermo scientific, 1:2000). For detection using this system, the membrane was first incubated with developing reagents (SuperSignal West Pico & West Femto), and then imaged using ImageQuant LAS 4000 (Life Sciences). Anti-HA-tag primary monoclonal antibody (M20003L, Abmart, 1:3000) was used to detect the expression of proteins in N. benthamiana leaves. Anti-GFP-tag primary monoclonal antibody (M20004L, Abmart, 1:3000) was used to detect the expression of SGP1 and its mutants in U. virens . Evans blue staining Evans Blue staining was performed to detect cell death in rice suspension cells [63] . This dye stains dead cells blue but does not stain living cells. The amount of Evans Blue released from rice suspension cells after staining was used as an indicator of cell death. Rice suspension cells were incubated with purified SGP1rec or MBP for 12 h followed by staining with 0.05% Evans Blue (Sigma) for 15 min. After extensive washing with water to remove excess dye, the blue dye taken up by dead cells was solubilized in 50% methanol with 1% SDS for 30 min at 50 °C and quantified by measuring light absorbance at 595 nm. VIGS assays in N. benthamiana pTRV1 and pTRV2:BAK1 plasmid constructs were introduced into Agrobacterium tumefaciens GV3101 by electroporation. The cultured Agrobacterium cells were harvested and resuspended in infiltration buffer (10 mM MgCl 2 , 10 mM MES, pH 5.7, and 150 mM acetosyringone) to an OD of 0.5. An Agrobacterium strain harboring the pTRV2:BAK1 vector and one harboring the pTRV1 vector were mixed in a 1:1 ratio and left in the dark at 28 °C for 2 h before infiltration into the lower leaf of a four-leaf stage N. benthamiana plant using a 1 mL needleless syringe. pTRV2:EV was used as a negative control, and the phytoene desaturase gene (PDS) was used to evaluate the effectiveness of the VIGS assay. At about 3 weeks post inoculation of pTRV strains, the third new leaves were collected for RNA extraction and RT-PCR analysis to validate the silencing efficiency. These leaves were albino in the TRV:PDS lines, and thus should exhibit silencing of the BAK1 gene in the TRV:BAK1 lines. Agrobacterium strains harboring elicitors were then infiltrated into the third new leaves of VIGS-silenced plants. Phase partition assay and PI-PLC treatment An HA tag was fused to the C terminus of the signal peptide and the N terminus of the mature SGP1 protein (SP-HA-mSGP1). The protein was expressed in N. benthamiana by Agrobacterium -mediated transient expression. Leaves were collected 2 days post Agro -infiltration. The protein was extracted with a homogenization buffer. After centrifugation for 10 min at 1200 × g and 4 °C, the post-nuclear supernatant was collected and phase partitioned with 2% (v/v) TX-114 according to a detailed protocol described previously [64] with minor modifications. The detergent phase was washed with Tris-buffered saline (TBS) three times and then incubated in the absence or presence of 2 U/mL PI-PLC for 1 h at 37 °C. The final aqueous and detergent fractions were analyzed by western blot with anti-HA antibody (M20003L, Abmart, 1:3000). To further test whether GPI modification was involved in the cell death activity of SGP1, PI-PLC (2 U/mL) was infiltrated into N. benthamiana leaves 24 h after Agro -infiltration, or PI-PLC was infiltrated into N. benthamiana leaves together with SGP1rec. Measurement of reactive oxygen species Reactive oxygen species (ROS) production was monitored with a luminol/peroxidase-based assay on leaf discs collected from 3- to 4-week-old N. benthamiana plants. The leaf discs were floated overnight in 200 μL of sterile H 2 O in a 96-well plate. H 2 O was replaced with working solution [luminol (35.4 μg/mL)/peroxidase (10 μg/mL) reaction solution supplied with sterile water and peptides at appropriate concentrations]. After the addition of the working solution, the plate was immediately moved to a GLOMAX96 microplate luminometer (Promega, Madison, WI, USA) for measurement of luminescence [24] . RNA extraction and RT-PCR analysis Total RNA was extracted using a NucleoSpin RNA II kit (Invitrogen) following the manufacturer’s instructions and treated with DNase I (TaKaRa) to remove DNA contamination. Approximately 800 ng of RNA was used for reverse transcription with oligo(dT) primers. Real-time PCR was performed using an SYBR Premix Ex Taq Kit II (TaKaRa) according to the manufacturer’s protocol. The relative quantitative method (2 −ΔΔCt ) was used to evaluate the quantitative variation [65] . The α- tubulin , NbEF1α , and Actin genes were used as internal controls for U. virens , N. benthamiana , and rice samples, respectively. MAPK assays Proteins were extracted from rice leaves and panicles after treatment with synthesized peptides using a plant phosphorylated protein extraction kit (HR0011, Baiaolaibo) following the manufacturer’s instructions. Phosphorylation of MAPK proteins was detected by immunoblotting with anti‐pMAPK antibody (#4370 s, Cell Signaling, 1:1000) and IRDye 800CW Goat anti-Rabbit IgG(H + L) antibody (926-32211, LI-COR, 1:10,000) according to the manufacturer’s protocol. Blots were stained with Ponceau S to verify equal loading. DAB staining N. benthamiana leaves were infiltrated with different peptides at a concentration of 1 μM. At 6 and 12 hpi, the infiltrated leaves were stained with 3,3-Diaminobenzidine (DAB, D8001, Sigma) solution for 8 h in the dark and then destained with ethanol before observation. Similarly, rice leaves and panicles incubated with different peptides were also stained with DAB at 6 or 12 hpi. Culturing of microbial strains and preparation of pathogen inocula Colonies of the U. virens WT strain and the transformants were grown on potato sucrose agar (PSA) medium plates. 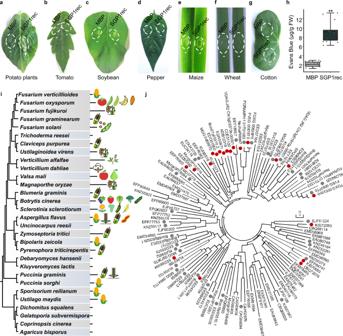Fig. 2: Specificity of the host response to SGP1 and wide distribution of SGP1 homologs across fungal species. a–hCell death responses in other plant species triggered by exposure to 1 μM SGP1rec or MBP control.a–gRepresentative leaves are shown for potato plants (a), tomato (b), soybean (c), pepper (d), maize (e), wheat (f), and cotton (g). Data were obtained from three independent experiments, with 10 plants of each species per experiment (Supplementary Data3). Dotted circles indicate infiltration area. The plus symbol (+) indicates that the cell death phenotype was observed, and the minus symbol (−) indicates the absence of a clear cell death phenotype.hCell death induced by SGP1rec in rice suspension cells. Cell death was quantified by detection of Evans Blue signal released from rice suspension cells (μg/g) after treatment with SGP1rec or MBP. Data were obtained from five independent experiments, with three replicates in each experiment. In box plots, whiskers indicate the minimum and maximum values, the line indicates the median, the box boundaries indicate the upper (25th percentile) and lower (75th percentile) quartiles. **P< 0.01, two-sidedt-test.iDistribution of SGP1 across fungal species. The fungal species include both plant pathogenic and non-pathogenic fungi. Left, Maximum-Likelihood phylogenetic tree of fungal species which contain the Ser-Thr-rich GPI-anchored domain, reconstructed using PhyML v3.0 based on single-copy orthologs (Supplementary Data5). Right, representative hosts of the corresponding pathogens. Image credit:https://www.flaticon.comorhttps://icons8.com/icons.jPhylogeny of SGP1 and 123 related sequences from selected fungal species (Supplementary Data2and4). The proteins that induce cell death inN. benthamianaare indicated by a red dot and those that do not are indicated by a gray dot. For conidia production, strains were cultured in PS liquid medium at 28 °C, with shaking at 150 rpm for 7 d. The cultures were then homogenized in a blender and adjusted to a concentration of about 10 6 conidia/mL for use as inoculum on rice. To prepare zoospores of P. parasitica , mycelia were cultured in 2.5% liquid V8 juice medium for 3 days and repeatedly washed with sterilized water at RT and incubated at 25 °C until sporangia formed. To initiate zoospore release, fresh cold water (4 °C) was added into the plates, which were then incubated at 4 °C. M. oryzae strains were cultured on complete medium agar plates at 28 °C. For conidia production of M. oryzae , strains were maintained on straw decoction and corn agar media at 28 °C for 7 days in the dark followed by 3 days of continuous illumination under fluorescent light [66] . Then, about 20 mL of sterilized water was poured into the plate and the conidia were collected using a paint brush. The conidia suspension was filtered through three layers of lens paper, and resuspended to a concentration of 5 × 10 4 spores/mL in sterile water. Xoo and B. glumae strains were grown on nutrient agar plates and King’s B medium plates at 28 °C for 2 days. Colonies were removed from the plate, washed twice, and resuspended to OD 600 = 0.8 in sterile distilled water for inoculation on rice. Transformation of U. virens The constructs for silencing the SGP1 gene or overexpressing SGP1 and its mutants were transformed into A. tumefaciens strain AGL-1 and then transformed into conidia of the U. virens WT strain using the ATMT method [67] , [68] , [69] . In brief, 100 μL of U. virens conidia (10 6 spores/mL) and 100 μL of A. tumefaciens strain AGL-1 containing the appropriate vector (OD600 was about 0.25) were mixed and spread on a nitrocellulose membrane. The nitrocellulose membrane was placed on a co-cultivation medium [69] plate for 3 days and then transferred onto 2% TB3 [0.3% yeast extract, 0.3% casamino acid, 1% glucose, 2% sucrose (w/v)], amended with hygromycin B (100 μg/mL) as a selection agent for transformants and cefotaxime (800 μg/mL) to counter-select bacteria. After incubation at 28 °C for 5–6 days, individual transformant colonies appeared and were transferred to PSA plates containing 100 μg/mL hygromycin B for the second round of selection. The silencing transformants were screened by qRT-PCR with primers SGP1-RT-F/R and UvTubulin1-F/R. UvTubulin1 was used to normalize the expression of SGP1 . The transformants overexpressing SGP1 were confirmed by western blot analysis with GFP antibody. Pathogenicity assays For assaying the pathogenicity of U. virens , during the booting stage (5–7 days before heading), 2 mL of inoculum was injected into the upper parts (5–7 cm from the upper node) of the swollen sheaths, which enclosed the developing panicles, of flag leaves on the main stem or main tiller using a syringe. The inoculum was injected into the space between the sheath and panicle to allow the inoculum to surround the spikelets. Disease symptoms were observed 30 days after inoculation. For inducing PR gene expression in rice using U. virens , detached leaves and panicles were immersed in the U. virens conidia for 6 h and then kept wet in a petri dish containing wet filter paper and incubated at 28 °C for another 6 h. For assaying the disease resistance triggered by synthesized peptides, N. benthamiana leaves, rice panicles, and rice leaves were pretreated with 1 μM peptide for 24 h before pathogen inoculation. The peptide was infiltrated into N. benthamiana leaves with a needleless syringe and, in rice, was syringe injected into the swollen sheaths of flag leaves on the main stems or main tillers, or was sprayed onto leaves. For P. parasitica inoculation, the detached leaves of 4-week-old N. benthamiana plants were inoculated with 100 zoospores of P. parasitica and kept on wet paper in a petri dish for 2 days in the dark at 25 °C. For M. oryzae inoculation, two-week-old rice seedlings were sprayed with 5 ×10 4 /mL spores of M. oryzae strain Guy11 and kept wet at 28 °C. Disease symptoms were observed 7 days after inoculation. The number of each type of lesion (0, no lesion; Type 1, pinhead-sized brown specks; Type 2, 1.5-mm brown spots; Type 3, 2–3-mm gray spots with brown margins; Type 4, many elliptical gray spots longer than 3 mm; Type 5, coalesced lesions infecting 50% or more of the leaf area) per 5 cm of leaf strip was scored. To determine the relative pathogen biomass in N. benthamiana , rice spikelets, and rice leaves, samples were collected at 24 hpi, 5 dpi, and 3 dpi, respectively. For Xoo inoculation on rice, rice leaves were cut with sterile scissors that had been dipped in a bacterial suspension of Xoo . For B. glumae inoculation on rice panicles, 2 ml of B. glumae inoculum was inoculated onto rice panicles in the same way as described for U. virens inoculation. Disease symptoms were measured at 7 dpi. The disease severity in rice panicles infected by B. glumae was evaluated using the following scale: 0, healthy panicle; 1, 0–20% diseased panicle; 2, 21–40% diseased panicle; 3, 41–60% diseased panicle; 4, 61–80% diseased panicle; 5, 81–100% diseased panicle. Disease severity was calculated using the following formula: disease severity = Σ (number of samples per rating × rating value)/total number of panicles. RNA sequencing profiling The mock- or SNP22-treated rice leaves and panicles were collected in three biological replicates. Samples from three biological replicates of the same treatment were pooled for RNA extraction and library preparation. After sequencing, clean reads were aligned to the Oryza sativa Japonica genome IRGSP-1.0 (Phytozome, http://www.phytozome.net ) using TopHat version 2.1.1 with default parameters. Clean reads and total mapped reads for each sample were shown on Supplementary Data 10 . Based on the length of each gene and the number of reads uniquely mapped to that gene, gene expression levels were normalized as fragments per kilobase of exon per million fragments mapped (FPKM) using Cufflinks version 2.2.1. To identify differentially expressed genes, a cutoff of |log2 fold change| (after adding “1” to each value in the matrix to avoid undefined values) > 2 was applied. The raw RNA-seq data have been deposited in the NCBI Sequence Read Archive data repository under accession number PRJNA690691. Confocal microscopy Conidia and mycelia were visualized using a confocal microscope (LSM 710; Carl Zeiss). Statistics and reproducibility SPSS statistics, GraphPad Prism, and Seaborn were used for data analysis. 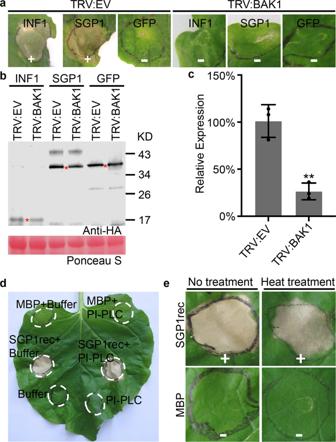Fig. 3: Cell death triggered by SGP1 requires BAK1 but is not affected after treatment with PI-PLC or heat inN. benthamiana. a–cCell death triggered by SGP1 requires BAK1.aSGP1-triggered cell death inTRV-silenced N. benthamiana. Representative photographs were taken at 5 days post-infiltration. Data were obtained from 3 independent experiments, each of which used 10 VIGS-silenced plants per line (Supplementary Data3). The plus symbol (+) indicates a positive cell death phenotype; minus symbol (−) indicates the absence of a clear cell death phenotype.bWestern blot analysis of proteins transiently expressed in VIGS-silencedN. benthamianaleaves. The red asterisks (*) indicate the predicted protein sizes.cqRT-PCR quantification of relative transcript levels ofBAK1in VIGS-silencedN. benthamianaleaves, normalized to those in TRV:EVlines, using theEF1αgene as an internal reference. Means and standard deviations obtained from three biological replicates. (**P< 0.01, two-sidedt-test).dCell death activity of SGP1rec in the presence or absence of PI-PLC, with MBP as a control. Data represent the results of three independent experiments in each of which one leaf was sampled and infiltrated from each of three plants per treatment (Supplementary Data3).eCell death response induced by heat-treated SGP1rec inN. benthamianaleaves. SGP1rec was treated under 100 °C for 10 min. Three independent experiments were performed (Supplementary Data3), in each of which ten leaves were sampled per treatment. The plus symbol (+) indicates a positive cell death phenotype; minus symbol (−) indicates the absence of a clear cell death phenotype. Similar results were obtained from three independent experiments in Figs. 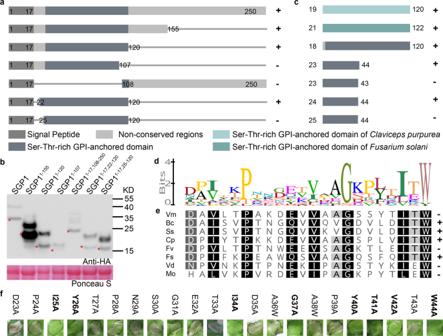Fig. 4: A 22 amino acid fragment in the N terminus of SGP1 is sufficient to mediate cell death inN. benthamiana. a–cRegions of SGP1 examined for cell death activity. Plus symbol (+), cell death phenotype; minus symbol (−), no clear cell death phenotype. Cell death phenotypes were recorded at 5 dpi.aRegions of SGP1 were examined for cell death activity by agrobacterium-mediated transient expression. Similar results were obtained from four independent experiments, with 10 plants per strain in each experiment (Supplementary Data3).bWestern blot analysis of SGP1 and truncated mutant variants transiently expressed inN. benthamianaleaves. The red asterisk (*) indicates the predicted protein sizes.cRegions of SGP1 examined for cell death activity inN. benthamianaby infiltration with 1 μM purified SGP1 variants fromE. coli. Similar results were obtained from three independent experiments (Supplementary Data3).dSequence logos indicating the level of conservation for each residue of SNP22 region in GPI-anchored proteins that trigger cell death from plant-associated fungi. Sequence logos were constructed with Geneious R11 (Supplementary Data6). The character and size of each logo represent the proportion of homologs with the amino acid at that specific site.e,fCell death triggered by expression of recombinant SNP22 homolog proteins from other fungi and alanine-substituted versions of SNP22rec.eSequence alignment and cell death-inducing activity of the SNP22 region of SGP1 homologs that can induce cell death. The homologous sequences of SNP22 from other fungi, including four amino acids flanking either terminus (Supplementary Data7), were expressed inE. coli.Vm, KUI59516 (Valsa mali);Bc, Bcin01p05310.2 (Botrytis cinerea);Ss, EDO01950 (Sclerotinia sclerotiorum);Cp, CCE31100 (Claviceps purpurea);Fv, FVEG_00876T0 (Fusarium verticillioides);Fs, NechaP98847 (Fusarium solani);Vd, VDAG_JR2_Chr3g03370a-00001 (Verticillium dahliae);Mo, MGG_04599T0 (Magnaporthe oryzae). Three independent experiments were performed, using 10 plants for each SNP22 homolog (Supplementary Data3) in each experiment.fRepresentative photos of cell death triggered by SNP22rec variants with single alanine substitutions at the indicated residues. Similar results were obtained from three independent experiments, with five plants per protein in each experiment (Supplementary Data3). 1 d, 7 c, and 8c as well as in Supplementary Figs. 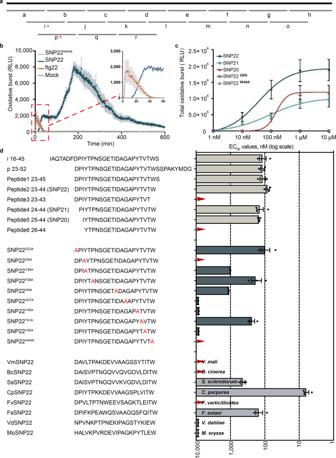Fig. 5: A 22 amino acid peptide (SNP22) of SGP1 is sufficient to induce ROS production inN. benthamiana. aSchematic representation of synthetic peptides (30-mer peptides, a–r) covering wild-type SGP1.bROS production dynamics induced by 1 μM peptides of SNP22 and SNP22W44AinN. benthamianaleaf discs. 100 nM flg22 and buffer served as positive and negative controls, respectively. ROS production was measured with a luminol-based assay. Leaf discs from 3- to 4-week-oldN. benthamianaplants were incubated with the indicated peptides, and the luminescence was expressed as relative light units (RLU). Values represent means ± SEM of three leaf disks, each sampled from a different plant and tested in parallel.cDose–response curves of total ROS production induced by SNP22, SNP21, SNP20, SNP22I25A, or SNP22W44Apeptides inN. benthamianaleaf discs. Values represent the means ± SEM of three independent experiments, each of which used three leaf disks per treatment.dSummary of EC50values determined from dose–response curves based on total ROS production. Peptide names and sequences are indicated on the left. EC50values of each peptide are shown on a logarithmic scale on the right. Values represent the means ± SEM of three independent experiments, with three leaf disks per treatment used in each experiment. No activity could be detected with peptides denoted by red triangles at 10 μM.Vm, KUI59516 (Valsa mali);Bc, Bcin01p05310.2 (Botrytis cinerea);Ss, EDO01950 (Sclerotinia sclerotiorum);Cp, CCE31100 (Claviceps purpurea);Fv, FVEG_00876T0 (Fusarium verticillioides);Fs, NechaP98847 (Fusarium solani);Vd, VDAG_JR2_Chr3g03370a-00001 (Verticillium dahliae);Mo, MGG_04599T0 (Magnaporthe oryzae). 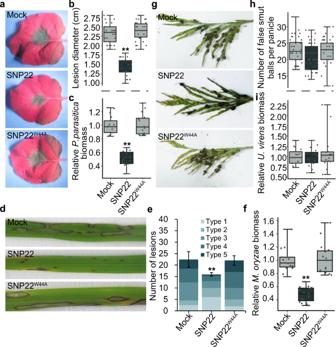Fig. 6: SNP22 triggers induction of disease resistance inN. benthamianaand rice. N. benthamianaleaves, rice panicles, and rice leaves were pretreated with 1 μM of the indicated peptide for 24 h before pathogen inoculation. Buffer served as a mock treatment. In box plots, whiskers indicate the minimum and maximum values, line indicates the median, the box boundaries indicate the upper (25th percentile) and lower (75th percentile) quartiles. (**P< 0.01 compared with Mock, two-sided Dunnett’s test).a–cInduction of disease resistance toP. parasitica var nicotianaeinN. benthamiana.aLesions were assessed under UV light and representative photographs were taken at 48 h post inoculation (hpi).bStatistical analysis of lesion diameters. Data was obtained from six independent experiments, each of which tested five leaves for each treatment.cRelative biomass ofP. parasiticainN. benthamianaleaves quantified by qPCR analysis of genomic DNA and normalized to mock treatment. Values from five biological replicates were shown, which include three technical replicates for each biological replicate.d–fInduction of disease resistance toM. oryzaein rice leaves.dRepresentative photographs were taken at 7 dpi.eQuantification of lesion types per 5 cm leaf strip. See Methods for description of lesion types. Values represent the means ± SD of five independent experiments, each of which used 10 leaves for each treatment.fRelative biomass ofM. oryzaein rice leaves, quantified by qPCR analysis of genomic DNA and normalized to mock treatment. Values from five biological replicates were shown, which include three technical replicates for each biological replicate.g–iDisease resistance toU. virensin rice panicles.gRepresentative photographs were taken at 30 dpi.hQuantification of false smut balls per panicle. The data were collected from five independent experiments, with a total of at least 44 panicles per line.iRelative biomass ofU. virensin rice spikelets, measured by qPCR analysis of genomic DNA and normalized to mock treatment. Values from five biological replicates were shown, which include three technical replicates for each biological replicate. 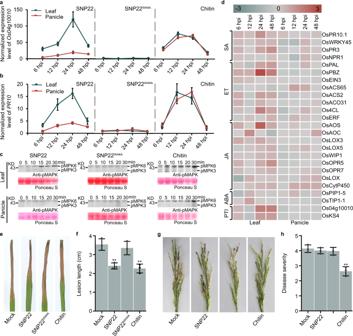Fig. 7: Immune responses triggered by SNP22 in rice leaves and panicles. a–cRice leaves and panicles were treated with either 1 μM SNP22 peptide, SNP22W44Apeptide, or chitin (hexa-N-acetylchitohexaose).a,bRelative induction of defense-related gene expression in rice leaves and panicles triggered by the indicated elicitors. Defense-related gene expression was normalized to that of mock at each time points after treatment. Riceactinserved as an internal reference. Values represent the means ± SEM of three biological replicates.cMAPK activation in rice leaves and panicles triggered by elicitors. The phosphorylation level of MAPK detected by immunoblot with anti-phospho-p44/42 MAPK (Erk1/2) antibody.dTranscriptome analysis. The relative gene expression was normalized to those of mock treatment at each time point post-treatment. Heatmap was shown based on lg values of the fold change. Cyan color, downregulation; red color, upregulation.e–hDisease resistance toX. oryzae pv. oryzaein rice leaves and toB. glumaein rice panicles triggered by the indicated elicitors. Rice leaves and panicles were pretreated with either 1 μM SNP22, SNP22W44A, or chitin 24 h before pathogen inoculation. Symptoms were assessed at 7 dpi. Three independent experiments were performed, and ten leaves or ten panicles were used for each experiment.eRepresentative photographs of symptoms on rice leaves caused byX. oryzae pv. oryzae.fLesion lengths. Values represent the means ± SD of three independent experiments, with ten leaves in each experiment (**P< 0.01 compared with Mock, two-sided Dunnett’s test).gRepresentative photographs of disease symptoms on rice panicles caused byB. glumae.hDisease severity in rice panicles, evaluated as described in the “Methods” section. Values represent the means ± SD of three independent experiments, with 10 panicles per treatment in each experiment (**P< 0.01 compared with Mock, two-sided Dunnett’s test). 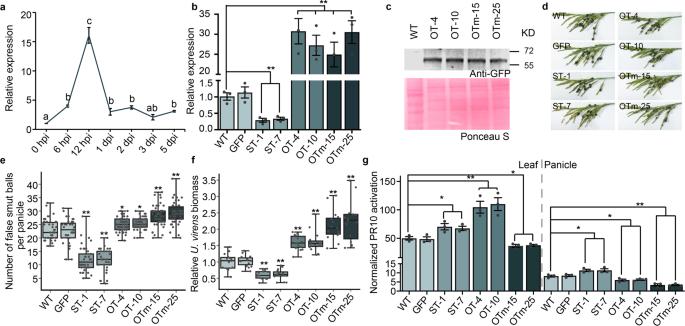Fig. 8: Involvement in pathogenicity and elicitor function of SGP1 duringU. virensinfection of rice panicles and challenge of rice leaves. aThe relative expression ofSGP1during different stages of infection.SGP1expression was normalized to its expression level prior to inoculation (0 hpi) usingTubulinas an internal reference. hpi, hours post inoculation; dpi, days post inoculation. Values are the means ± SEM of three biological replicates. The different letters indicate statistically significant differences (P< 0.05) as measured by Duncan’s multiple range test.bRelative transcript levels ofSGP1in differentU. virenstransgenic lines. The transcript levels were measured by qRT-PCR and normalized to those in the WT strain usingTubulinas an internal reference. ST,SGP1-silenced transformants ofU. virens; OT,SGP1overexpression transformants ofU. virens; OTm,SGP1W44Aoverexpression transformants ofU. virens. Values are the means ± SEM of three biological replicates. (**P< 0.01; two-sidedt-test).cWestern blot analysis of SGP1 and SGP1W44AinU. virensWT and transgenic lines with anti-GFP antibody.d–fPathogenicity phenotypes of transgenicU. virenslines and WT. In box plots, whiskers indicate minimum and maximum values, line indicates the median, the box boundaries indicate the upper (25th percentile) and lower (75th percentile) quartiles.dRepresentative photographs of disease symptoms on rice panicles.eQuantification of the number of false smut balls per panicle. Data were collected from five independent experiments, with a total of at least 31 panicles per line. (*P< 0.05; **P< 0.01 compared with WT, two-sided Dunnett’s test).fRelativeU. virensbiomass in infected spikelets, measured by qPCR of genomic DNA and normalized to WT. Values from five biological replicates were shown, which include three technical replicates for each biological replicate. (**P< 0.01 compared with WT, two-sided Dunnett’s test).gRelative induction ofPR10transcription in rice leaves and panicles at 12 hpi. The induction of PR10 expression inU. virens-inoculated rice was normalized to that in mock-inoculated rice, withActinserving as an internal reference. Values are the means ± SEM of three biological replicates. (**P< 0.01; *P< 0.05; two-sidedt-test). 1 , 3 a, and 11c, d. Reporting summary Further information on research design is available in the Nature Research Reporting Summary linked to this article.